Species-specific defence responses facilitate conspecifics and inhibit heterospecifics in above–belowground herbivore interactions Conspecific and heterospecific aboveground and belowground herbivores often occur together in nature and their interactions may determine community structure. Here we show how aboveground adults and belowground larvae of the tallow tree specialist beetle Bikasha collaris and multiple heterospecific aboveground species interact to determine herbivore performance. Conspecific aboveground adults facilitate belowground larvae, but other aboveground damage inhibits larvae or has no effect. Belowground larvae increase conspecific adult feeding, but decrease heterospecific aboveground insect feeding and abundance. Chemical analyses and experiments with plant populations varying in phenolics show that all these positive and negative effects on insects are closely related to root and shoot tannin concentrations. Our results show that specific plant herbivore responses allow herbivore facilitation and inhibition to co-occur, likely shaping diverse aboveground and belowground communities. Considering species-specific responses of plants is critical for teasing apart inter- and intraspecific interactions in aboveground and belowground compartments. A growing body of research shows that aboveground and belowground herbivores can affect each other and shape community structure [1] , [2] , [3] , [4] . Plants can mediate these interactions through the production of primary and secondary compounds and reallocation of these chemicals between shoots and roots [5] , [6] , [7] , [8] , [9] . Most of these studies have focused on interspecific aboveground and belowground herbivore interactions [10] , [11] , [12] , and some studies have examined interactions of aboveground and belowground herbivores that are different life stages of the same species [13] , [14] , [15] . However, the very small number of studies comparing inter- and intraspecific aboveground and belowground herbivore interactions that often occur simultaneously in nature do not currently allow reliable prediction of the outcome of such interactions [10] , [16] , [17] , [18] . These interactions, which could be facilitation, inhibition or both, may determine herbivore population dynamics, preventing species dominance and maintaining a diversity of shoot- and root feeders, and subsequently affecting community and ecosystem stability. In a system with multiple herbivores feeding on shoots and roots, variation in herbivore types may determine the outcome of aboveground and belowground interactions because of plant specificity in response to herbivory [10] , [11] , [12] . Increasing evidence shows that chewing herbivores mainly induce plant defences through a jasmonic acid-mediated response and sucking herbivores mainly induce a salicylic acid-mediated response [19] , [20] . Therefore, these different herbivore feeding modes may contribute to variation in plant defence responses, which can change the pattern of resource and secondary chemical allocation between aboveground and belowground compartments [11] , [21] . However, the prediction that herbivores within a feeding guild will have stronger or more consistently negative interactions has little support in the literature [18] . Moreover, plants may differ in their responses to specialist versus generalist herbivores both through induction of different responses by generalists and specialists or the prevention of a secondary chemical response that could increase the performance of chemical sequestering specialists [22] , [23] . However, plant responses to specialists versus generalists may not be consistent and distinct enough to allow diet breadth to predict the outcome of interactions [22] , [23] . In addition to herbivore feeding modes and their diet breadth, plant responses may potentially be more specific with aboveground and belowground herbivore identities [16] , [17] . If herbivores are different life stages of the same species that facilitate each other’s performance, this may boost or maintain their populations on the shared host plant. In contrast, negative conspecific effects may limit herbivore populations through negative feedbacks as plants are increasingly frequently attacked by both life stages. Positive conspecific effects would favour coexistence of life stages by speeding competitive exclusion of other species, whereas negative conspecific effects may enhance other species’ coexistence by limiting the dominance of the species with multiple life stages that attack the same plant. On the other hand, heterospecific aboveground and belowground herbivores may inhibit each other by competing for shoot and/or root resources or by changing plant defences [24] , [25] , [26] but they may also enhance each others’ performance through increases in resources and/or reduction in defences [5] , [27] . Thus, species-specific plant responses to herbivores may dramatically affect aboveground and belowground herbivore population dynamics and community composition [10] , [11] , [12] . To date, however, studies on aboveground and belowground interactions including multiple shoot and root herbivores that vary with feeding mode, diet breadth and species identities are rare [16] , [17] . Here we investigate herbivore interactions with a plant, Triadica sebifera (Euphorbiaceae), that is attacked by several aboveground insect species including a species of specialist flea beetle, Bikasha collaris (Coleoptera: Chrysomelidae), which has both a aboveground adult and belowground larval life stage. As one of the major components of aboveground insect communities, adults of many beetles feed on plant leaves, whereas their larvae live underground feeding on roots. Plants bearing these conspecific adults and larvae are often attacked by other aboveground herbivores such as caterpillars, weevils and aphids, providing an ideal system for studying inter- and intraspecific aboveground and belowground herbivore interactions. Our previous studies show that B. collaris adults facilitate larval performance, whereas larvae inhibit adult survival and these interactions are mediated by plant shoot and root chemicals [13] , [28] . However, we know little about how these conspecific interactions are affected by co-occurring heterospecific herbivores and how the plant responds to these various types of aboveground and belowground herbivory. As inhibition is more common than facilitation between heterospecifics [18] , in this study, we predict that heterospecific aboveground herbivores will inhibit B. collaris larvae and, in turn, belowground herbivory effects on heterospecific aboveground herbivores will be consistently negative. We also predict that plants will show species-specific responses to herbivory and these responses will mediate insect interactions through chemical defence. Specifically, we asked following questions: (i) Do the effects of conspecific flea beetle adults on belowground larvae reflect a general plant response to aboveground herbivory or a more specific plant response related to herbivore feeding mode and/or diet breadth? (ii) How does the presence of belowground larvae affect conspecific and heterospecific aboveground insect species feeding and abundance? (iii) What is the role of plant secondary chemicals in these conspecific and heterospecific aboveground and belowground interactions? We report laboratory and field data demonstrating that facilitation and inhibition of aboveground and belowground herbivores co-occur. We show that these interactions depend on species identity: although conspecific aboveground adults increased belowground larval survival and abundance, heterospecific aboveground insects inhibited belowground larvae or had no effect. Belowground larvae reduced abundance of conspecific adults and of heterospecifics but increased conspecific feeding. These ecological effects as well as the variation in aboveground and belowground herbivore performances are closely related to changes in tannin concentrations in shoots and roots. These findings will improve our understanding of the mechanisms that determine aboveground and belowground species coexistence and community assembly. Experiment 1: effects of aboveground B. collaris adults and heterospecific insects on belowground B. collaris larvae Effects of aboveground herbivory on survival of belowground B. collaris larvae depended on aboveground herbivore identity (F 6,49 =11.75, P <0.0001; one-way analysis of variance (ANOVA), n =56; Fig. 1a ). Relative to undamaged plants ( Fig. 1a , ‘N’), aboveground B. collaris adult feeding increased conspecific belowground larval survival more than 65% ( Fig. 1a , ‘Bc’). In contrast, heterospecific aboveground chewing by the other Coleoptera ( Fig. 1a , ‘SC’) and Lepidoptera ( Fig. 1a , ‘SL’ and ‘GL’) significantly inhibited belowground B. collaris larval survival. Aboveground herbivory by phloem sucking Hemiptera ( Fig. 1a , ‘GH’) or mechanical damage ( Fig. 1a, ‘M ’) did not affect belowground larval survival. 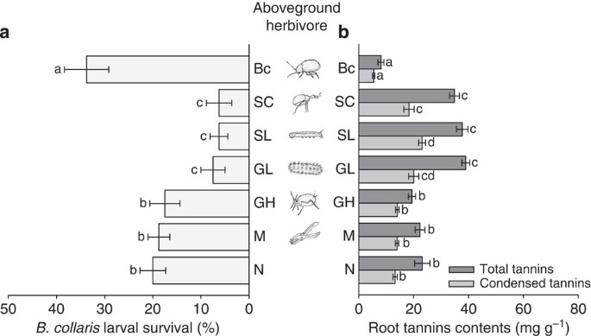Figure 1: Effects of conspecific and heterospecific aboveground herbivory on belowground insects and root chemical. (a)B. collarislarval survival and (b)T. sebiferaroot tannins (dark grey bars, total tannins; light grey bars, condensed tannins) in Experiment 1 (multiple herbivore species experiment). Aboveground herbivory treatments: Bc,B. collarisadult; GH, generalist aphid (Hemiptera,Aphissp.); GL, generalist caterpillar (Lepidoptera,C. flavescens); M, Mechanical; N, none (undamaged controls) ; SC, specialist weevil (Coleoptera,H. bicallosicollisis); SL, specialist caterpillar (Lepidoptera,G. inexacta). Values are means+1 s.e. (n=56). Same letters indicate means that were not significantly different inpost-hoctests for each response variable. Figure 1: Effects of conspecific and heterospecific aboveground herbivory on belowground insects and root chemical. ( a ) B. collaris larval survival and ( b ) T. sebifera root tannins (dark grey bars, total tannins; light grey bars, condensed tannins) in Experiment 1 (multiple herbivore species experiment). Aboveground herbivory treatments: Bc, B. collaris adult; GH, generalist aphid (Hemiptera, Aphis sp. ); GL, generalist caterpillar (Lepidoptera, C. flavescens ); M, Mechanical; N, none (undamaged controls) ; SC, specialist weevil (Coleoptera, H. bicallosicollisis ); SL, specialist caterpillar (Lepidoptera, G. inexacta ). Values are means+1 s.e. ( n =56). Same letters indicate means that were not significantly different in post-hoc tests for each response variable. Full size image Aboveground herbivores significantly affected root total tannins (F 6,49 =38.19, P <0.0001; one-way ANOVA, n =56) and condensed tannins (F 6,49 =22.39, P <0.0001; one-way ANOVA, n =56), but did not change total phenolics (F 6,49 =2.17, P =0.062; one-way ANOVA, n =56). Relative to undamaged plants, aboveground B. collaris adults significantly decreased root total and condensed tannins ( Fig. 1b ). In contrast, heterospecific aboveground chewing herbivores (Coleoptera and Lepidoptera) significantly increased root total and condensed tannins ( Fig. 1b ). Aphids (Hemiptera) and mechanical damage did not significantly affect root total or condensed tannins ( Fig. 1b ). Experiment 2: field interactions between aboveground herbivores and belowground B. collaris larvae Survival of belowground B. collaris larvae depended on types and amounts of damage. Leaf damage by B. collaris adults correlated positively with conspecific belowground larval survival ( Fig. 2a ). However, leaf damage by heterospecific Lepidoptera insects correlated negatively with belowground B. collaris larval survival ( Fig. 2b ). In a multiple regression with both damage type and block, larval survival increased with B. collaris adult damage (F 1,79 =33.11, P <0.0001; coefficient=+8.5% survival per % damage; regression analysis, n =90), decreased with Lepidoptera insect damage (F 1,79 =30.72, P <0.0001; coefficient=−4.3% survival per % damage; regression analysis, n =90), but did not depend on block (F 8,79 =1.88, P =0.0742; regression analysis, n =90). 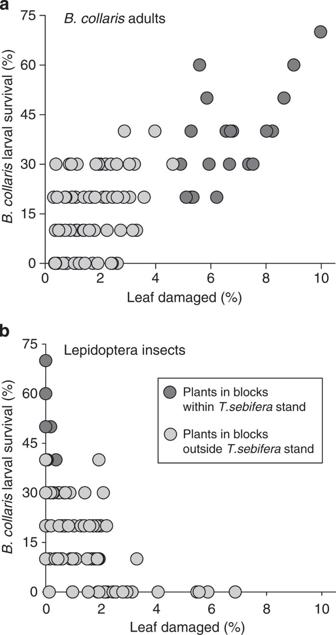Figure 2: Insect identity andB. collarisadults abundance affectB. collarislarval survival. (a) conspecificB. collarisadults damage and (b) heterospecific Lepidoptera insects damage in blocks located inside (dark circles) or outside (light circles) of theT. sebiferastand in Experiment 2 (field experiment). Figure 2: Insect identity and B. collaris adults abundance affect B. collaris larval survival. ( a ) conspecific B. collaris adults damage and ( b ) heterospecific Lepidoptera insects damage in blocks located inside (dark circles) or outside (light circles) of the T. sebifera stand in Experiment 2 (field experiment). Full size image In surveys, B. collaris adults were the most abundant herbivores on T. sebifera plants, with small numbers of Lepidoptera insects ( Supplementary Table 1 , Supplementary Fig. 1 ) including G. inexacta , G. geometrica , P. litura , B. marginata , C. flavescens as well as a single H. bicallosicollisis (Coleoptera) and Aphis sp. (Hemiptera). There were fewer B. collaris adults ( Table 1 , Fig. 3a ) but more leaf damage ( Table 1 , Fig. 3b ) on plants with conspecific belowground larval herbivory than those without larvae. The abundance of ( Table 1 , Fig. 3c ) and leaf damage from ( Table 1 , Fig. 3d ) Lepidopterans decreased with belowground larval presence. However, total leaf damage did not depend on B. collaris larval herbivory ( Table 1 ). All these factors varied with experimental block and time ( Table 1 , Supplementary Figs 2,3 ). Table 1 Repeated ANOVA analyses of belowground B. collaris larvae effects on conspecific and heterospecific aboveground insect abundance and leaf damage. 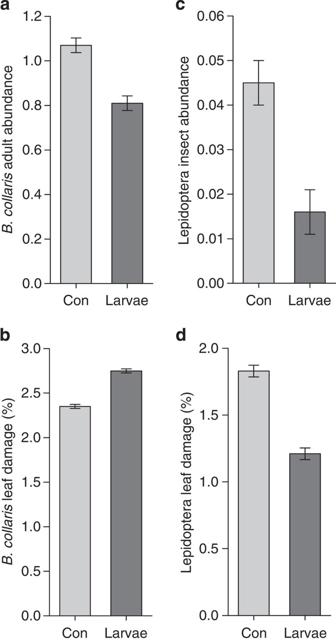Figure 3: Effects of belowgroundB. collarislarval herbivory on aboveground herbivore abundance and damage. (a)B. collarisadult abundance, (b) percent leaf area damaged byB. collarisadults, (c) Lepidoptera insect abundance and (d) percent leaf area damaged by Lepidoptera insects in Experiment 2 (field experiment). Belowground herbivory treatments: Con, undamaged controls; Larvae,B. collarislarvae herbivory. Values are means+1 s.e. (n=90). Full size table Figure 3: Effects of belowground B. collaris larval herbivory on aboveground herbivore abundance and damage. ( a ) B. collaris adult abundance, ( b ) percent leaf area damaged by B. collaris adults, ( c ) Lepidoptera insect abundance and ( d ) percent leaf area damaged by Lepidoptera insects in Experiment 2 (field experiment). Belowground herbivory treatments: Con, undamaged controls; Larvae, B. collaris larvae herbivory. Values are means+1 s.e. ( n =90). Full size image Experiment 3: phenolic compounds as the mediator of aboveground adults and belowground larvae of B. collaris Survival of larvae and adults were both higher on US plants with lower phenolic concentrations than on Chinese plants with higher concentrations ( Table 2 , ‘Origin’, Fig. 4 ). Adult feeding significantly increased larval survival and decreased condensed tannins ( Supplementary Fig. 4a ), total tannins ( Fig. 4a ) and total phenolics ( Fig. 4b ) in the roots ( Table 2 , ‘Adults’), and these effects were stronger on US plants than on Chinese plants ( Table 2 , ‘Origin × Adults’). In contrast, larval feeding significantly decreased adult survival and increased condensed tannins ( Supplementary Fig. 4b ) and total tannins ( Fig. 4c ), but not total phenolics ( Fig. 4d ) in the leaves ( Table 2 , ‘Larvae’). Adult survival was not affected by the interaction of plant origin and larvae ( Table 2 , ‘Origin × Larvae’). Table 2 ANOVAs analysing the effects of plant origin, herbivory and their interaction on conspecific herbivore survival and phenolic compounds. 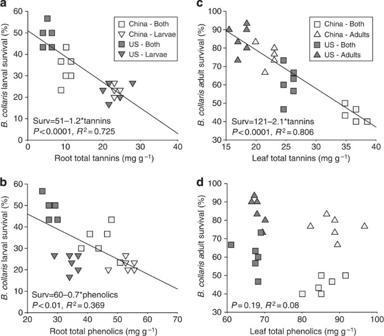Figure 4: Relationship betweenB. collarissurvival and phenolic compounds in roots and leaves. Left: regression of larval survival on root (a) total tannins and (b) total phenolics; right: regression of adult survival on leaf (c) total tannins and (d) total phenolics in Experiment 3 (population experiment). Triangles pointing down indicate plants with only larvae, triangles pointing up indicate plants with only adults and squares indicate plants with both larvae and adults. Dark symbols indicate plants from populations in the United States. Light symbols indicate plants from populations in China. Lines,P-values andr-values are from reduced major axis (RMA) regressions. Full size table Figure 4: Relationship between B. collaris survival and phenolic compounds in roots and leaves. Left: regression of larval survival on root ( a ) total tannins and ( b ) total phenolics; right: regression of adult survival on leaf ( c ) total tannins and ( d ) total phenolics in Experiment 3 (population experiment). Triangles pointing down indicate plants with only larvae, triangles pointing up indicate plants with only adults and squares indicate plants with both larvae and adults. Dark symbols indicate plants from populations in the United States. Light symbols indicate plants from populations in China. Lines, P -values and r -values are from reduced major axis (RMA) regressions. Full size image Regressions indicated that larval survival was negatively affected by increasing root condensed tannins ( Supplementary Fig. 4a ), total tannins ( Fig. 4a ) and total phenolics ( Fig. 4b ). However, adult survival was only negatively affected by increasing leaf condensed tannins ( Supplementary Fig. 4b ) and total tannins ( Fig. 4c ), but not leaf phenolics ( Fig. 4d ). There were few significant effects of experimental factors in ANOVAs with regression residuals ( Table 2 ). Our study reports plant-mediated interactions of conspecific and heterospecific aboveground and belowground herbivores. We show that these interactions depend on species identity: although conspecific aboveground adults increased belowground larval survival and abundance, heterospecific aboveground insects inhibited belowground larvae (chewers) or had no effect (sucking or mechanical damage). The positive effect of conspecific feeding could not be explained as simply an effect of diet breadth (other specialists had negative effects), feeding mode (other chewers had negative effects) or taxonomic order (other Coleoptera had negative effects). Also, presence of belowground larvae increased conspecific adults’ feeding, whereas decreasing heterospecific insects’ feeding and abundance. All of these ecological effects (positive and negative; direction of effect (aboveground on belowground, belowground on aboveground)) as well as the variation in aboveground and belowground herbivore performances feeding on different T. sebifera populations are consistent with changes in tannin concentrations in shoots and roots. Our results reveal reciprocal effects between conspecific and heterospecific species in aboveground and belowground compartments. The positive effects of B. collaris adults on larval survival ( Figs 1 and 2 ) and the presence of larvae on adult feeding ( Fig. 3 ) suggest that conspecific aboveground and belowground herbivores can magnify their impacts on host plants, but the negative effect of larvae on adult abundance ( Fig. 3 ) and survival ( Fig. 4 ) makes it difficult to predict the net effects on population sizes. However, the negative effects of heterospecific aboveground herbivores on B. collaris larvae may limit the dominance of B. collaris ( Figs 1 and 2 ). These contrasting patterns were clearly shown by the higher larval survival in blocks in the Triadica stand (with more B. collaris adults) than in blocks outside the Triadica stand (with less B. collaris adults) in our field study ( Fig. 2 ). On the other hand, the negative effects of B. collaris larvae on heterospecific aboveground herbivores may reduce their impact on larvae if this influences the feeding choices of aboveground herbivores. The limited mobility of larvae prevents them from choosing to feed on other plants in response to aboveground herbivory, whereas more mobile aboveground herbivores may choose to feed on plants without larvae if they can tell whether larvae are present. These results demonstrate that conspecific facilitation and heterospecific inhibition can co-occur between the aboveground and belowground compartments, which may improve our understanding the role of inter- and intraspecific aboveground and belowground herbivore interactions in regulating population dynamics and community diversity. Studies, such as ours, that simultaneously compare inter- and intraspecific aboveground and belowground herbivore interactions may add a new dimension to studies on species interactions, in particular for those in which some species have aboveground and belowground feeding life stages. As predictions of the outcome of inter- and intraspecific interactions of folivorous insects may not apply to cases with both aboveground and belowground herbivores [18] , considering belowground species and their interactive effects with aboveground species are especially important to understanding the intra- versus interspecific aboveground interactions in a community having belowground insects. For example, a recent study reported that the effects of belowground root larvae of the fly Delia radicum on aboveground community members varied depending on species identity, with an increasing oviposition of adult fly on the plant infested by its larvae [17] . In our study system, as B. collaris adults and larvae feed on leaves and roots, respectively, their interactions with heterospecific aboveground insects are likely to differ substantially from the example of the fly D. radicum whose adults lay eggs on the host plant but consume nectar. These few studies point to challenge of understanding how species-specific responses from host plants mediate the interactions between conspecific and heterospecific insects, especially those that are spatiotemporally separated and so do not directly interact. In this study, we found that herbivory by aboveground weevils and caterpillars significantly inhibited B. collaris larval survival, whereas aphid feeding and mechanical damage had no effects, indicating specific responses of plants to aboveground herbivory determine belowground insect performance. Our study was unreplicated in terms of sucking feeders (only the single aphid species) but the difference between this species and all chewing herbivores provides some support for herbivore feeding mode driving plant responses [18] . However, we found the wide variation in plant responses to different specialists or different generalists and similar responses to some generalists and specialists suggests limited utility in using diet breadth as a predictor of plant responses for this plant species. Indeed, the range of plant responses we observed highlights the need to have replication in testing the effects of herbivore feeding mode, diet breadth or taxonomy on plant defence responses. Our chemical analyses suggest that the observed conspecific and heterospecific aboveground and belowground herbivore interactions may be mediated by plant secondary chemicals. Phenolics such as tannins are considered especially important in defence against specialist insects as digestibility-reducing compounds [29] , [30] . Moreover, studies have shown that plants with different tannin content may support different insect communities [29] , [31] , [32] . In our study, positive or negative interactions between insects were closely related to decreases or increases, respectively, in tannin concentrations in leaves (for aboveground herbivore survival) or roots (for larval survival). Indeed, the independence of residuals from regressions of tannins and survival from ANOVA factors in Experiment 3 is strong support for tannins playing a major role in the variation in B. collaris survival among T. sebifera populations and herbivore conditions. Together, the results of these three experiments indicate that variation in the quantity and distribution of these secondary chemicals is closely related to aboveground–belowground herbivore interactions among multiple herbivores at ecological and evolutionary time scales. Tannins vary in their defence against insects, in part depending insect gut pH [30] , [33] . However, in this study, we measured condensed tannins, total tannins and total phenolics; thus further chemical analyses and bioassays are needed to identify the specific tannin compounds that affect B. collaris survival. In addition, allocation of primary compounds, such as nitrogen, between shoots and roots may also affect aboveground and belowground insect development [7] , [13] . The mother-knows-best hypothesis states that parents maximize the survival and performance of their offspring by preferentially ovipositing on high nutrition or low resistance plants [34] , [35] . Our results may extend this hypothesis that adults facilitate larval performance not only by preferential oviposition, but also possibly by their feeding, which decreases secondary chemical defences to benefit larvae. In this study, adult feeding decreased tannin content in the roots, which likely facilitated larvae survival, as indicated by the significant negative relationship between root tannin content and larval survival. Given that heterospecific insect feeding can increase tannins in T. sebifera roots and negatively affect larvae, increasing tannin levels in the leaves (from larval root feeding) might interfere with leaf feeding by heterospecific insects, thereby indirectly facilitating larval survival. Sequence of arrival is considered important in determining plant-mediated interactions between herbivores, especially for herbivores with one generation per year because early season feeders have a greater potential to affect later feeders [10] , [12] , [18] , [36] . Thus, the natural sequence of herbivory events may play an important role in determining the interactions between aboveground and belowground herbivores [4] , [37] . But, these effects may be more complicated for herbivores with overlapping generations. In this study system, B. collaris passes through at least five generations from May to October in our study area. During most of this period, the multivoltine moths, aphids and weevils we tested are all also active. Thus, these aboveground and belowground herbivores often occur simultaneously and our results in Experiments 1 and 2 likely reflect their interactions under natural conditions. In summary, our study shows that induced changes in defences facilitate conspecifics and inhibit heterospecifics in the interactions of aboveground–belowground herbivores with multiple feeding types. These findings will improve our understanding of the mechanisms that determine aboveground and belowground species coexistence and community assembly. The varying secondary chemicals in and different performance of insects on plant populations suggest changes in plant chemical defence may affect aboveground and belowground herbivore communities. Our results will also have important implications for pest insect management and biological control of invasive plants using conspecific aboveground and belowground insects [36] , [38] , as these insects are often considered to be important agricultural and forest pests, or promising biocontrol agents to fight invasive plants if they are host specific. The interactive effects involved in systems with multiple aboveground and belowground herbivores that vary in feeding modes and species identities are complex, considering species-specific responses of plants may help to tease apart those inter- and intraspecific interactions. Study system Triadica sebifera (Euphorbiaceae) is a rapidly growing tree native to Asia and invasive in the United States of America [39] . Triadica sebifera supports a diversity of herbivores in China ( Supplementary Fig. 1 ) [40] . For example, Bikasha collaris (Coleoptera: Chrysomelidae) is a T . sebifera specialist flea beetle with leaf-feeding adults and root-feeding larvae [41] . Heterapoderopsis bicallosicollisis (Coleoptera: Attelabidae) is a specialist weevil with leaf-chewing adults, and larvae that feed in rolled leaf structures called nidi [42] . Lepidoptera whose caterpillars attack this tree include generalists such as Cnidocampa flavescens (Limacodidae), Grammodes geometrica (Noctuidae), Prodenia litura (Noctuidae) and Biston marginata (Geometridae) and the specialist Gadirtha inexacta (Noctuidae) [43] . In addition, generalist Aphis sp. (Homoptera: Aphididae) feed on T. sebifera phloem [40] . All these leaf-feeders are among the most abundant and damaging insects and commonly feed concurrently with belowground B. collaris larvae on T. sebifera from July to September in the Wuhan, China ( Supplementary Fig. 1 ). Thus, these insects used in this experiment are most representative of the natural composition of herbivore assemblages on T. sebifera in the study area. Plants and insects We used T. sebifera seeds from a natural population near Wuhan, China (31°33′N, 114°07′E), for Experiments 1 and 2 and seeds from six populations across southern China and six populations across the southeastern United States for Experiment 3 ( Supplementary Table 2 ). We planted seeds in an unheated greenhouse at Wuhan Botanical Garden, Hubei, China (30°32′N, 114°24′E). After 4 weeks, when plants had four or five leaves, we transplanted them individually into pots filled with topsoil (collected from a local field without T. sebifera ) and grew them in an unheated greenhouse with ambient temperature and humidity and natural light until the start of each experiment. For belowground herbivory, we obtained B. collaris eggs by having adults lay eggs in Petri dishes following Huang et al. [28] . For aboveground herbivores, we collected nidi of H. bicallosicollisis and larvae of G. inexacta and C. flavescens from a field in Wuhan, reared them on local T. sebifera plants under laboratory conditions (26–30 °C, 50–70% relative humidity, 14:10 h light : dark photoperiod), and used their offspring for experiments. We collected B. collaris adults and Aphis sp. aphids from sites in Wuhan for experiments. Experiment 1: effects of aboveground B. collaris adults and heterospecific insects on belowground B. collaris larvae To test the effects of conspecific and heterospecific aboveground herbivory on belowground B. collaris larval survival, we used aboveground treatments of damage by adults of B. collaris, H. bicallosicollisis and Aphis sp., and larvae of G. inexacta and C. flavescens , as well as mechanical damage and an undamaged control ( Supplementary Fig. 1 ). The aboveground herbivores studied included representatives of three orders (Coleoptera (2 species), Lepidoptera (2) and Hemiptera (1)), two types of host ranges (specialist (3) and generalist (2)) and two feeding guilds (leaf chewer (4) and phloem feeder (1)). Six weeks after transplantation (day 0), we selected similarly sized plants (height: 23.9±0.4 cm, stem diameter: 2.61±0.04 mm, number of leaves: 16.9±0.3) and transferred ten newly laid B. collaris eggs onto the roots of each plant following Huang et al. [28] . Then, we enclosed each plant in a nylon mesh cage (100 cm high, 20 cm diameter) and arranged plants randomly within eight rows in an unheated greenhouse. Within each row, we randomly assigned two plants to each of the seven aboveground herbivory treatments (2 replicates × 7 herbivory treatments, 14 plants in each row, 16 replicates in total). Rows were 1 m apart and plants within each row were 0.3 m apart from each other. Row did not explain any response variable and is not included in analyses. To make aboveground and belowground herbivory occur simultaneously, we imposed aboveground herbivory treatments on day 9 when B. collaris eggs were hatching and left aboveground herbivores on the plants for 18 days, which is the average larval development time [41] . To make aboveground and belowground herbivory experimentally independent, we sealed the nylon mesh cage of each pot using string attached to the plant stem below all leaves. For conspecific aboveground herbivory, we added ten B. collaris adults to the leaves of each plant. Previous studies reported that ten adults removed approximately ten percent of the leaf area in 18 days when ten larvae of B. collaris attacked the plant simultaneously [41] . To reduce confounding effects of damage level on belowground B. collaris larval performance, we also selected ten percent of leaf area removed for the damage level of heterospecific aboveground herbivory treatments. For H. bicallosicollisis herbivory, we added two newly emerged male adults to each plant and replaced individuals that died during the experiment. For caterpillar herbivory, we added one first-instar G. inexacta larva or two first-instar C. flavescens larvae to each plant, because per capita feeding rate of G. inexacta is higher than that of C. flavescens [44] . We replaced larvae of G. inexacta and C. flavescens with new first-instar ones every 4 and 3 days, respectively, as late instars of both species can quickly cause severe damage, which would exceed the 10% target for defoliation. For herbivory by Aphis sp., we placed 50 adult aphids on each plant. This density is consistent with average abundance observed for the same size of aphids attacking plants in the field (51.7±3.1 aphids per plant, n =60). For mechanical damage, we punched seven to nine holes (diameter 0.6 cm) into randomly selected leaves of each plant every day. The quantity and timing of leaf area removed by mechanical damage coincided with real herbivory treatments. We did not manipulate control plants. On day 27, we removed all aboveground herbivores and visually estimated the leaf area removed from each plant. There were no significant differences in leaf area removed among aboveground herbivory treatments (F 4,75 =1.22, P =0.31; one-way ANOVA, n =80; excluding aphid herbivory treatment and control). We harvested 8 of the 16 plants from each treatment and analysed condensed tannin, total tannin and total phenolic concentrations in the roots. We observed and removed B. collaris adults emerging from the soil on the remaining eight plants every day. Experiment 2: field interactions between aboveground herbivores and belowground B. collaris larvae To further examine the effects of conspecific and heterospecific aboveground herbivory on belowground B. collaris larval survival under natural conditions, as well as the effects of belowground B. collaris larvae herbivory on aboveground herbivore communities, we conducted a manipulative experiment in a field at Wuhan Botanical Garden. In this field, there was a 5-year-old T. sebifera stand (about 240 plants), with 1 m spacing between plants. Plants in the stand were heavily damaged by abundant B. collaris adults and had some damage from specialist, H. bicallosicollisis and G. inexacta, and generalist, C. flavescens and Aphis sp. The stand was surrounded by various vegetable crops and herbs (typical of environments where T. sebifera occurs naturally in China), which were attacked by generalist insects, including C. flavescens , G. geometrica , B. marginata , P. litura and Aphis sp. ( Supplementary Fig. 1 ). To examine the effects of B. collaris adult abundance on larval survival, we established nine blocks (1 × 1 m) in the field that varied in distance to the T. sebifera stand and were presumably exposed to a gradient of B. collaris adult abundance. Two blocks were 7 m apart in the centre of the T . sebifera stand colonized by B. collaris . Seven blocks were outside of the T . sebifera stand with each an additional 8 m away from the stand. Blocks were plowed and sprayed twice with herbicide before the start of the experiment. Ten weeks after, seedlings were transplanted (day 0), 20 pots with similarly sized plants (stem height: 31.0±0.3 cm, stem diameter: 3.48±0.04 mm, number of leaves: 29.4±0.4) were buried 15 cm deep in the soil in each block (five rows of four plants). We added belowground herbivores (ten newly laid B. collaris eggs per plant—see above) to ten randomly chosen pots in each block and left the other ten pots as controls (damaged plants neighbouring control ones). To prevent oviposition by adults into the soil of pots but allow the aboveground plant parts (leaves and stems) to be exposed to naturally occurring herbivores, we enclosed the belowground parts of each plant with mesh. To examine the effects of belowground B. collaris larvae on conspecific and heterospecific aboveground herbivores, we visually checked all leaves on each plant and recorded the identity and abundance of insects on all plants ( n =180) every 3 days over a period of 36 days, since belowground B. collaris development time including egg, larva and pupa is about 36 days [41] . Meanwhile, we also visually estimated leaf area damaged by B. collaris or caterpillars to the nearest 5% every 3 days. B. collaris adult feeding produces irregular pits and scars, whereas caterpillar feeding on leaves produces large irregular holes or skeletonized leaves. Damage made by H. bicallosicollisis is similar to that of B. collaris adults. We only found one H. bicallosicollisis during the field survey and so assumed all irregular pits and scars were due to B. collaris in our analyses. To determine the effects of conspecific and heterospecific aboveground herbivores on belowground B. collaris larvae, we counted the number of B. collaris adults emerging from the soil for plants that received belowground herbivores ( n =90). Experiment 3: phenolic compounds as the mediator of aboveground and belowground herbivores To test whether changes in phenolic compounds might be the causal mechanism underlying aboveground and belowground herbivore interactions, we assayed phenolic compounds in leaves and roots of different T. sebifera ecotypes after attack by larvae and/or adults of B. collaris . Previous studies reported that plants from China have higher tannin levels than their US counterparts [44] , [45] , [46] . Therefore, this experiment was structured as a 2 × 2 × 12 full factorial design incorporating two levels of aboveground herbivory (0 versus 10 adults per plant), two levels of belowground herbivory (0 versus 10 eggs per plant), 12 T. sebifera populations (six per range, Supplementary Table 2 ) and six replicates. Six weeks after transplantation (day 0), we selected similarly sized plants, enclosed each in a nylon mesh cage, and randomly assigned four plants of each population to each of six rows in an unheated greenhouse with the same spacing as in Experiment 1. Row did not explain any response variable and is not included in analyses. We randomly assigned one plant of each population in each row to one of the four different herbivory treatments. The timing of herbivory treatments was the same as in Experiment 1. At the end of the herbivory treatment period (day 27), we harvested three plants of each treatment combination and analysed condensed tannin, total tannin and total phenolic concentrations in leaves and roots (three replicates). For remaining plants, we recorded the number of surviving B. collaris adults on plants subjected to aboveground herbivory treatments and removed them, and counted the number of adults emerging from the soil of plants with belowground herbivores daily (three replicates). Chemical analyses We dried leaves and roots of each plant separately at 40 °C for 5 days. We ground samples in a ball mill then stored them at −20 °C in sealed plastic bags before chemical analyses. We extracted samples (100 mg) with 1 ml of 70% (v/v) acetone (1 h, room temperature), sonicated them (20 min), and then, removed insoluble material by centrifugation (5 min, 10,000 r.p.m., 4 °C). We estimated condensed tannin content using the acid butanol assay [45] , [47] by mixing leaf extracts (0.5 ml) with 6 ml of butanol-HCl reagent ( n -butanol/concentrated HCl, 95:5, v/v) and 0.2 ml of iron reagent (2% FeNH 4 (SO 4 ) 2 ·12 H 2 O in 2 N HCl), oven heating mixtures (100 °C, 60 min), cooling them to room temperature and measuring their absorbance at 550 nm. We used commercial cyanidin chloride (Sigma-Aldrich) as a standard. We estimated total tannin content using a radial diffusion assay [48] by placing leaf extracts (40 μl) in 5 mm diameter holes in 1% (wt/v) agarose plates with 0.1% (wt/v) BSA, incubating plates (30 °C, 96 h) and measuring precipitated protein area. We used commercial tannic acid (Sigma-Aldrich) as a standard. We estimated total phenolic content using the modified prussian blue assay [49] . We mixed sample extracts (100 μl) with 3 ml distilled water, 1 ml of 0.016 M K 3 Fe(CN) 6 and 1 ml of 0.02 M FeCl 3 . After 15.0 min, we added 5 ml of stabilizer (0.2% Gum Arabic in 17% H 3 PO 4 ) and measured absorbance at 700 nm. We used commercial Gallic Acid Monohydrate (Sigma-Aldrich) as a standard. All chemical concentrations are expressed as mg g −1 dry weight. Data analyses For Experiment 1, we used one-way ANOVAs to analyse the impacts of aboveground herbivores on belowground B. collaris larval survival and phenolic compounds in roots. We used Student–Newman–Keuls post-hoc tests for multiple comparisons among treatments. For Experiment 2, we performed separate regression analyses to determine the relationships between belowground B. collaris larval survival and leaf area damaged by conspecific or heterospecific herbivory. We calculated leaf area damaged per plant by averaging across surveys. We analysed the impact of belowground B. collaris larval herbivory on the abundance and leaf area damaged by conspecific and heterospecific herbivores separately using repeated measures ANOVAs (fixed effect: larval herbivory, block; time: 11 level categorical variable). For Experiment 3, we used two-way ANOVAs to analyse the impact of herbivory and plant origin on belowground B. collaris larval survival and root phenolic compounds (three fixed effects, origin, adult herbivory and their interaction), and on aboveground B. collaris adult survival and leaf phenolic compounds (three fixed effects, origin, larval herbivory and their interaction). Plant populations (six populations per range) were nested within origin as the random effect. We performed separate regression analyses to determine the relationship between insect survival and phenolic compounds. To examine the role of changes in phenolic compounds in the effects of experimental treatments on survival in the ANOVAs, we performed regressions of survival on phenolic compounds and examined the dependence of regression residuals on experimental treatments in follow-up ANOVAs. In these analyses, significant effects in survival and chemical ANOVAs along with a significant regression result and a lack of a significant effect in the residual ANOVA indicates survival responses are strongly related to chemical changes. We performed all data analyses with SAS, version 9.1 (SAS Institute). How to cite this article: Huang, W. et al. Species-specific defence responses facilitate conspecifics and inhibit heterospecifics in above–belowground herbivore interactions. Nat. Commun. 5:4851 doi: 10.1038/ncomms5851 (2014).